Intracellular temperature mapping with a fluorescent polymeric thermometer and fluorescence lifetime imaging microscopy Cellular functions are fundamentally regulated by intracellular temperature, which influences biochemical reactions inside a cell. Despite the important contributions to biological and medical applications that it would offer, intracellular temperature mapping has not been achieved. Here we demonstrate the first intracellular temperature mapping based on a fluorescent polymeric thermometer and fluorescence lifetime imaging microscopy. The spatial and temperature resolutions of our thermometry were at the diffraction limited level (200 nm) and 0.18–0.58 °C. The intracellular temperature distribution we observed indicated that the nucleus and centrosome of a COS7 cell, both showed a significantly higher temperature than the cytoplasm and that the temperature gap between the nucleus and the cytoplasm differed depending on the cell cycle. The heat production from mitochondria was also observed as a proximal local temperature increase. These results showed that our new intracellular thermometry could determine an intrinsic relationship between the temperature and organelle function. Temperature is a fundamental physical quantity that governs every biological reaction within living cells [1] , [2] , [3] , [4] . The biological reactions responsible for cellular functions occur either exothermically or endothermically at particular locations within a cell, such as inside organelles. Thus, temperature distributions inside a living cell reflect the thermodynamics and functions of cellular components [5] . In medical studies, the cellular pathogenesis of diseases (for example, cancer) is characterized by extraordinary heat production [6] . Therefore, intracellular temperature mapping of living cells should promote better understanding of cellular events and the establishment of novel diagnoses and therapies [7] . In spite of the considerable demand and expectation in various fields of life science, intracellular temperature distributions within living cells have not yet been observed, because no thermometry was capable of intracellular temperature mapping. First of all, conventional thermometers (that is, thermography and thermocouples) have low spatial resolution (up to 10 μm) and are unable to function within cells. In contrast to conventional thermometers, fluorescent molecular thermometers [8] , [9] , [10] , [11] , [12] are promising tools for intracellular thermometry, as they function at the molecular level. Nevertheless, when considered as a tool to observe intracellular temperature distribution, the fluorescent molecular thermometers should simultaneously satisfy multiple requirements, that is, high temperature resolution, high spatial resolution, functional independency of environmental changes in pH and ionic strength, as well as functional independency of surrounding biomacromolecules, and concentration-independent output. The unavailability of these features has been an obstacle to intracellular temperature mapping. For example, we created a fluorescent nanogel thermometer (FNT) by combining a thermo-responsive polymer with a water-sensitive fluorophore in addition to intensive developments of the fluorescent molecular thermometer over the past few years [13] , [14] , [15] , [16] , [17] , [18] , [19] , [20] , [21] . As we reported in a previous paper, FNT functioned even in living cells and showed high sensitivity to changes in temperature, thus enabling intracellular thermometry with high temperature resolution (better than 0.5 °C in the range between 27 and 33 °C) [22] . However, FNT could measure only the average temperature of the whole cell. It could not reveal any intracellular temperature distribution, because the relatively large size (62 nm or more in hydrodynamic diameter) and low hydrophilicity (aggregation was induced at temperatures higher than 27 °C) of FNT hindered the dispersion of this temperature probe throughout the cell. In this study, we developed a novel fluorescent polymeric thermometer (FPT) that could diffuse throughout the cell and applied it to intracellular temperature mapping, where the fluorescence lifetime of FPT was adopted as a temperature-dependent variable. In intracellular temperature mapping, the fluorescence lifetime permits an accurate measurement of temperature, because it is independent of fluctuations under experimental conditions, such as the concentration of FPT at a given location within a cell or the strength of the excitation source. Specifically, time-correlated single photon counting (TCSPC) system-based fluorescence lifetime imaging microcopy (FLIM) [23] was used in our intracellular thermometry to measure the temperature-dependent fluorescence lifetime of FPT with the highest accuracy [24] . Our new thermometric methodology using FPT and TCSPC-FLIM had a high spatial and temperature resolution. This method was sufficient to perform temperature mapping in living cells in which novel biological insights, such as intracellular temperature gradients and organelle-specific thermogenesis, were unequivocally revealed. Fluorescent polymeric thermometer To create a fluorescent molecular thermometer that would diffuse throughout a living cell, we prepared an upgraded FPT ( Fig. 1a , M n =19,300, M w / M n =2.1) of a reduced size (8.9 nm in hydrodynamic diameter in the globular state, Supplementary Fig. S1 ) and with sufficiently hydrophilic residues. FPT works using an established temperature-sensing mechanism ( Fig. 1b ) [25] , [26] , [27] . At low temperatures, a thermo-responsive poly- N - n -propylacrylamide (NNPAM) sequence in FPT assumes an extended structure with hydration of amide linkages, in which a water-sensitive N -{2-[(7- N , N -dimethylaminosulfonyl)-2,1,3-benzoxadiazol-4-yl](methyl)amino}ethyl- N -methylacrylamide (DBD-AA) unit can be quenched by neighbouring water molecules. At higher temperatures, which weaken hydration, the polyNNPAM sequence shrinks because of the hydrophobic interaction among the NNPAM units, resulting in the release of water molecules and strong fluorescence from the DBD-AA unit. Additionally, an ionic potassium 3-sulfopropyl acrylate (SPA) unit enriches the hydrophilicity of FPT to prevent interpolymeric aggregation within a cell. 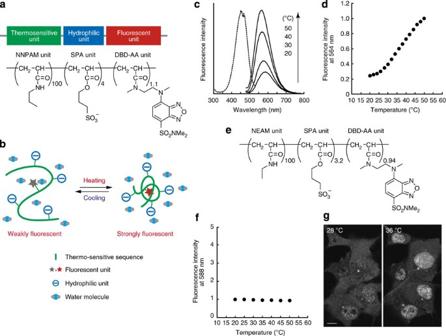Figure 1: FPT for intracellular temperature mapping. (a) Chemical structure. The original name of each unit is described in the main text. (b) Functional diagram in an aqueous medium. (c) Fluorescence spectra in a COS7 cell extract. An excitation spectrum (broken, at 30 °C) was obtained from emissions at 565 nm and normalized. Emission spectra (solid) were obtained with an excitation at 456 nm. (d) Fluorescence intensity response to the temperature variation in a COS7 cell extract. The fluorescence quantum yield was 0.25 at 50 °C. (e) Chemical structure of the control copolymer. (f) Relationship between the fluorescence intensity of the control copolymer in a COS7 cell extract (excited at 456 nm) and the temperature. (g) Confocal fluorescence images of FPT in living COS7 cells. Scale bar represents 10 μm. Figure 1: FPT for intracellular temperature mapping. ( a ) Chemical structure. The original name of each unit is described in the main text. ( b ) Functional diagram in an aqueous medium. ( c ) Fluorescence spectra in a COS7 cell extract. An excitation spectrum (broken, at 30 °C) was obtained from emissions at 565 nm and normalized. Emission spectra (solid) were obtained with an excitation at 456 nm. ( d ) Fluorescence intensity response to the temperature variation in a COS7 cell extract. The fluorescence quantum yield was 0.25 at 50 °C. ( e ) Chemical structure of the control copolymer. ( f ) Relationship between the fluorescence intensity of the control copolymer in a COS7 cell extract (excited at 456 nm) and the temperature. ( g ) Confocal fluorescence images of FPT in living COS7 cells. Scale bar represents 10 μm. Full size image The fluorescence properties of FPT were examined using a COS7 cell extract. Complementary experiments indicated that the COS7 cell extract had an environment that was nearly identical to the interior of living COS7 cells ( Supplementary Fig. S2 ). As shown in Fig. 1c, d , FPT showed stronger fluorescence in a COS7 cell extract in accordance with temperature increases. This fluorescence response was independent of ionic strength (in the range of 0.1–0.2) and environmental pH (6–10; Supplementary Fig. S3 ) at values that include the ranges of physiological variations in the cytosol [28] , [29] . A control copolymer without thermosensitivity ( Fig. 1e, f , M n =15,100, M w / M n =2.6) was also prepared. The only difference in chemical structure between FPT and the control copolymer is the methylene chain length of the major unit (that is, 3 and 2, respectively). The diminished hydrophobicity of the control copolymer renders itself extended even at high temperatures in an aqueous solution. Aside from the response to temperature, its structural similarity to FPT ensured comparable behaviour in living cells. To examine the intracellular distribution of FPT, it was microinjected into the cytoplasm of COS7 cells, and the resulting fluorescence images were recorded using a confocal fluorescence microscope. The obtained fluorescence images of the COS7 cells ( Fig. 1g ) showed that regardless of temperature, FPT could diffuse throughout the cells (both within the nucleus and in the cytoplasm). This distribution of FPT throughout the entire cell suggested the feasibility of intracellular mapping with high spatial resolution. Fluorescence lifetime as a temperature-dependent parameter As shown in Fig. 1g , we found that the fluorescence intensity of FPT was higher in the nucleus than in the surrounding cytoplasm; this difference in intensity was significant when the temperature of the medium was 36 °C. The observed difference in intensity between the nucleus and cytoplasm could reflect the distribution of intracellular temperatures, but a difference in probe concentration between the two compartments would also considerably influence the fluorescence intensity. Therefore, the fluorescence lifetime (an index of the relaxation time from the excited state), which is independent of concentration [30] , was adopted as a temperature-dependent variable of FPT for the imaging of intracellular temperature. The fluorescence lifetime measurements of FPT in a COS7 cell extract indicated that the fluorescence decay curves consisted of two exponential components ( Fig. 2a ). From the previous photophysical study on a copolymer labelled with DBD-AA units [30] , it can be affirmed that fast and slow fluorescence decays of FPT originated from the hydrogen-bonded and the hydrogen bond-free DBD-AA units, respectively. Thus, the fluorescence lifetime of FPT was calculated with the measured coefficients of the double-exponential function (see Methods ). In a COS7 cell extract, the fluorescence lifetime of FPT was prolonged as the solution temperature increased ( Fig. 2b , closed circle), and was shortened as the solution temperature decreased ( Supplementary Fig. S4 ). Moreover, this fluorescence lifetime response of FPT was not sensitive to either the variation in probe concentration ( Fig. 2c ), the surrounding proteins ( Supplementary Fig. S5 ) or environmental viscosity ( Supplementary Fig. S6 ). The relationship between the fluorescence lifetime of FPT in COS7 cell extracts and temperature ( Fig. 2b , closed circle) was used as a calibration curve for temperature imaging. The temperature resolution in the thermometry of the COS7 cells was evaluated to be 0.18–0.58 °C within the range of 29–39 °C ( Fig. 2b , open circle). In contrast to FPT, the fluorescence lifetime of the control copolymer showed a complete lack of sensitivity to temperature variation ( Fig. 2d ). 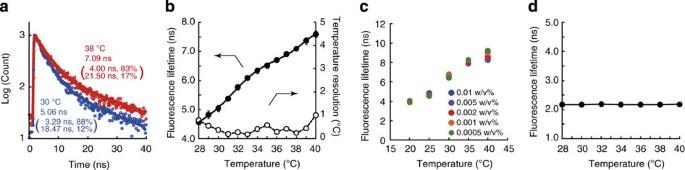Figure 2: Temperature-dependent fluorescence lifetime of FPT. (a) Representative fluorescence decay curves of FPT in a COS7 cell extract. The fluorescence lifetime and its two components are also indicated. (b) Calibration curve (closed, left axis) and temperature resolution (open, right axis) of FPT. (c) Concentration independence of FPT in COS7 cell extracts. (d) Relationship between the fluorescence lifetime of the control copolymer in a COS7 cell extract and temperature. Figure 2: Temperature-dependent fluorescence lifetime of FPT. ( a ) Representative fluorescence decay curves of FPT in a COS7 cell extract. The fluorescence lifetime and its two components are also indicated. ( b ) Calibration curve (closed, left axis) and temperature resolution (open, right axis) of FPT. ( c ) Concentration independence of FPT in COS7 cell extracts. ( d ) Relationship between the fluorescence lifetime of the control copolymer in a COS7 cell extract and temperature. Full size image In performing TCSPC-FLIM on living COS7 cells, the fluorescence decay curve of FPT at each pixel was obtained with high repeatability unless the experimental conditions (for example, sample and temperature) were changed, and was a double-exponential function at every pixel within the cells. Then, the fluorescence lifetime at each pixel was calculated from the corresponding double-exponential function ( Supplementary Fig. S7 ), which allowed the construction of fluorescence lifetime images. The fluorescence lifetime of each pixel within the COS7 cells was prolonged with increased culture medium temperature ( Fig. 3a, b ). It should be noted that we have confirmed that the fluorescence signal in fluorescence lifetime images was derived from FPT, not from auto-fluorescence of living cells ( Supplementary Fig. S8 ). Moreover, the temperature-dependent change in fluorescence lifetime was not observed when the control copolymer was used ( Fig. 3c, d ). The fluorescence lifetime images of living COS7 cells with FPT ( Fig. 3a ) had larger deviations in fluorescence lifetime (5.3–5.7%) than those of a COS7 cell extract containing FPT ( Supplementary Fig. S9 ) (1.9–2.1%), indicating that intracellular temperature distribution takes place within the living COS7 cells. Related fluorescence lifetime images of a dividing COS7 cell were also successfully obtained with FPT (and the control copolymer; Supplementary Fig. S10 ). From these results, it can be concluded that the fluorescence lifetime is a suitable variable in intracellular temperature mapping using the novel sensor FPT. 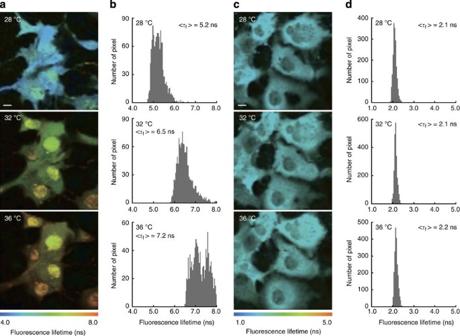Figure 3: Temperature imaging of living COS7 cells by TCSPC-FLIM with FPT. (a, b) Fluorescence lifetime images of FPT (a) and histograms of fluorescence lifetime in whole living cells (b). (c,d) Fluorescence lifetime images of the control copolymer (c) and histograms of fluorescence lifetime in whole living cells (d). The temperatures indicated in the images were of the culture medium. <τf>represents an average of the histogram. Scale bar represents 10 μm. Figure 3: Temperature imaging of living COS7 cells by TCSPC-FLIM with FPT. ( a, b ) Fluorescence lifetime images of FPT ( a ) and histograms of fluorescence lifetime in whole living cells ( b ). ( c , d ) Fluorescence lifetime images of the control copolymer ( c ) and histograms of fluorescence lifetime in whole living cells ( d ). The temperatures indicated in the images were of the culture medium. < τ f >represents an average of the histogram. Scale bar represents 10 μm. Full size image Imaging of the intracellular temperature distributions Next, the temperature distributions in living COS7 cells were investigated with a particular focus on organelles. It is noteworthy that the energy of glucose metabolism in cells is equivalent to a temperature increase of at least 2 °C within an entire cell, because of the following reasons: the total free energy released by the oxidation of glucose (glucose +6O 2 →6CO 2 +6H 2 O) is 2870 kJ mol −1 ; the specific heat capacity of the cell can be estimated to be 4.184 J (gK) −1 (similar to water); the intracellular glucose concentration is kept to at least 3–5 mM, when the culture medium includes 25 mM glucose (that is, in the present condition) [31] . This encouraged us to utilize FPT (with a temperature resolution of 0.18–0.58 °C) for intracellular temperature imaging. We set the temperature of the culture medium to ca. 30 °C, the temperature at which a specimen can readily and consistently be maintained due to only a small difference from the ambient temperature (ca. 24–27 °C). Biological activities such as cell proliferation were confirmed at this temperature. Culture medium of higher temperature (for example, 37 °C) resulted in a larger error of fluorescence lifetime of FPT within the imaging field, most likely due to the considerable temperature gap between the optical set-up in the microscope and the sample, which unignorably reduced the accuracy of intracellular thermometry (cf. maximum errors in determining temperature within the imaging field at 30 and 37 °C are 0.35 and 1.3 °C, respectively). By performing TCSPC-FLIM on living COS7 cells containing FPT ( Fig. 4a ), we attributed the heterogeneous fluorescence intensities of COS7 cells (as discussed in the previous section) to the temperature differences inside the cell. 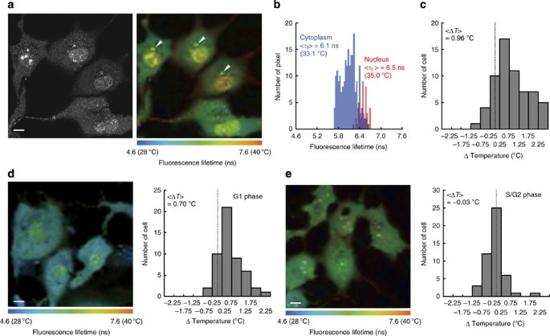Figure 4: Temperature mapping in living COS7 cells. (a) Confocal fluorescence image (left) and fluorescence lifetime image (right) of FPT. (b) Higher temperature in the nucleus. Histograms of the fluorescence lifetime in the nucleus and in the cytoplasm in a representative cell (the leftmost cell ina). The s.e. in determining a temperature was 0.38 °C. (c) Histogram of the temperature differences between the nucleus and the cytoplasm (n=62). ΔTemperature was calculated by subtracting the average temperature of the cytoplasm from that of the nucleus. <ΔT> represents an average of the histogram. (d,e) Cell-cycle-dependent thermogenesis in the nucleus. Representative fluorescence lifetime images and histograms of ΔTemperature in living cells synchronized to G1 phase (n=51) (d) and S/G2 phase (n=48) (e). The potential maximum error in determining ΔTemperature value was 0.35 °C. In (a–e), the temperature of the medium was maintained at 30 °C. Scale bar represents 10 μm. Figure 4: Temperature mapping in living COS7 cells. ( a ) Confocal fluorescence image (left) and fluorescence lifetime image (right) of FPT. ( b ) Higher temperature in the nucleus. Histograms of the fluorescence lifetime in the nucleus and in the cytoplasm in a representative cell (the leftmost cell in a ). The s.e. in determining a temperature was 0.38 °C. ( c ) Histogram of the temperature differences between the nucleus and the cytoplasm ( n =62). ΔTemperature was calculated by subtracting the average temperature of the cytoplasm from that of the nucleus. <Δ T > represents an average of the histogram. ( d , e ) Cell-cycle-dependent thermogenesis in the nucleus. Representative fluorescence lifetime images and histograms of ΔTemperature in living cells synchronized to G1 phase ( n =51) ( d ) and S/G2 phase ( n =48) ( e ). The potential maximum error in determining ΔTemperature value was 0.35 °C. In ( a – e ), the temperature of the medium was maintained at 30 °C. Scale bar represents 10 μm. Full size image The most notable feature of the resultant temperature distributions is the difference in temperature between the nucleus and the cytoplasm, as observed in numerous cells. In a representative cell, the temperature of the nucleus, evaluated from the fluorescence lifetime at each pixel in the image, was significantly higher than that of the cytoplasm ( Fig. 4b ). Analysis of many cell samples ( n =62) revealed that the average temperature difference between the nucleus and the cytoplasm was 0.96 °C ( Fig. 4c ). This thermal pool in the nucleus may originate from its activities, such as DNA replication, transcription and RNA processing, as well as its structural separation by the nuclear membrane [32] . Strikingly, we found that this temperature gap between the nucleus and cytoplasm was dependent on the cell cycle: the nucleus was warmer (by 0.70 °C on average) in cells synchronized to the G1 phase ( Fig. 4d ), whereas there was little temperature gap in S/G2-phased cells ( Fig. 4e ). It is likely that this temperature homogeneity at the S/G2 phase was the result of a temperature increase in the cytoplasm rather than a temperature decrease in the nucleus. Consistent with our results, this cell-cycle-dependent heat production was previously observed from a mass of cells in a study using a microcalorimeter [33] . Another remarkable feature of the temperature imaging ( Fig. 4a ) was a single spot in the perinuclear region (arrowheads). This spot, observed in 56% of the cells imaged, was identified as a centrosome by co-localization with γ-tubulin ( Fig. 5a ). Temperature imaging with FPT by TCSPC-FLIM revealed that the centrosome is also significantly warmer (by 0.75 °C on average) than the cytoplasm, with considerable cell-to-cell variation ( Fig. 5b ). This centrosome-specific thermogenesis might be associated with its diverse functions, such as mitosis and the organization of microtubules [34] . The hydrolysis of tubulin GTP, ATP-driven motion of motor proteins (for example, dynein and kinesin), and phosphorylation/dephosphorylation of centrosomal proteins by kinase/phosphatase are all possible heat source at the centrosome [35] . 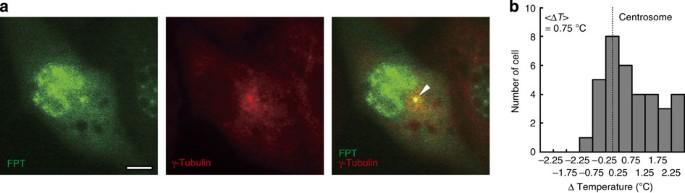Figure 5: Heat production from the centrosome in living COS7 cells. (a) Heat production near the centrosome (arrowhead). Epifluorescence images of FPT (left), the centrosome visualized with γ-tubulin antibody (middle) and their merged image (right). (b) Histogram of temperature differences between the centrosome and the cytoplasm (n=35). ΔTemperature was calculated by subtracting the average temperature of the cytoplasm from that of the centrosome with the potential maximum error of 0.35 °C. The temperature of the medium was maintained at 30 °C. Scale bar represents 10 μm. Figure 5: Heat production from the centrosome in living COS7 cells. ( a ) Heat production near the centrosome (arrowhead). Epifluorescence images of FPT (left), the centrosome visualized with γ-tubulin antibody (middle) and their merged image (right). ( b ) Histogram of temperature differences between the centrosome and the cytoplasm ( n =35). ΔTemperature was calculated by subtracting the average temperature of the cytoplasm from that of the centrosome with the potential maximum error of 0.35 °C. The temperature of the medium was maintained at 30 °C. Scale bar represents 10 μm. Full size image Imaging of local thermogenesis at mitochondria Finally, we studied the local heat production by mitochondria. Mitochondria release surplus energy in the form of heat through respiration. To image this local thermogenesis, the temperature distribution and locations of the mitochondria were co-visualized by FPT and a mitochondria indicator, respectively ( Fig. 6a ). The enlarged fluorescence lifetime image clearly showed localized thermogenesis near the mitochondria ( Fig. 6a , arrowheads). It is notable that this mitochondria-mediated heat production was supported by the intracellular distribution of our previous nanogel thermometer FNT ( Supplementary Figs S11 and S12 ). As described in our previous paper [22] , FNT inside living COS7 cells moderately aggregates at culture medium temperatures greater than 27 °C ( Supplementary Fig. S11a ). Considering that the aggregation of FNT is triggered by heat, it probably began at the warmest place within the cytosol. To determine the location of aggregated FNT, representative organelles (that is, mitochondria, lysosomes, endoplasmic reticulum (ER) and the Golgi apparatus) were co-visualized. As a result, aggregated FNT was found to reside near mitochondria ( Supplementary Fig. S11b, c ), but not near other organelles, including lysosomes, ER and the Golgi apparatus ( Supplementary Fig. S12 ). Thus, it could be concluded that the local temperature near the mitochondria is higher than the temperature of the rest of the space in the cytosol (aside from the centrosome). 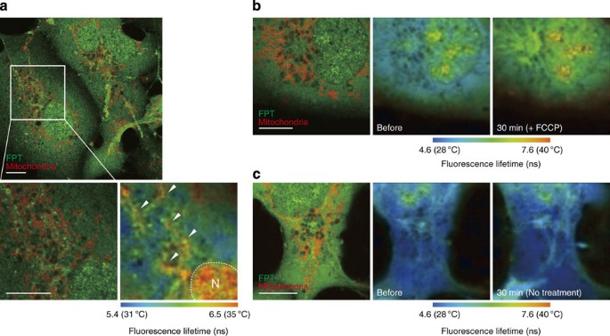Figure 6: Local heat production near the mitochondria in living COS7 cells. (a) Confocal fluorescence images of FPT (green) and MitoTracker Deep Red FM (red; upper and left lower) and fluorescence lifetime image of FPT (right lower). The region of interest, as shown in the square in the upper panel, is enlarged in the lower panels. Arrowheads point to local heat production. In the right lower panel, N indicates the nucleus. (b) Temperatures increase near the mitochondria after the inhibition of ATP synthesis by the uncoupler FCCP. Confocal fluorescence images of FPT (green) and MitoTracker Deep Red FM (red; left) and fluorescence lifetime images of FPT (middle and right). (c) Control experiment for (b) No significant change in the fluorescence lifetime of FPT was detected without a chemical stimulus. In (a–c), the temperature of the medium was maintained at 30 °C. Scale bar represents 10 μm. Figure 6: Local heat production near the mitochondria in living COS7 cells. ( a ) Confocal fluorescence images of FPT (green) and MitoTracker Deep Red FM (red; upper and left lower) and fluorescence lifetime image of FPT (right lower). The region of interest, as shown in the square in the upper panel, is enlarged in the lower panels. Arrowheads point to local heat production. In the right lower panel, N indicates the nucleus. ( b ) Temperatures increase near the mitochondria after the inhibition of ATP synthesis by the uncoupler FCCP. Confocal fluorescence images of FPT (green) and MitoTracker Deep Red FM (red; left) and fluorescence lifetime images of FPT (middle and right). ( c ) Control experiment for ( b ) No significant change in the fluorescence lifetime of FPT was detected without a chemical stimulus. In ( a–c ), the temperature of the medium was maintained at 30 °C. Scale bar represents 10 μm. Full size image Furthermore, this local heat release from the mitochondria is accelerated when ATP synthesis is stalled by an uncoupling reagent [36] . Thus, a temperature increase due to local heat production from the mitochondria following the addition of an uncoupling reagent, 4-(trifluoromethoxy)phenylhydrazone (FCCP) [37] , was imaged in FPT-filled COS7 cells ( Fig. 6b, c ). As evaluated from fluorescence lifetime images of whole COS7 cells, this heat production by FCCP resulted in an average temperature increase of 1.02±0.17 °C (avg.±s.d., n =7) inside COS7 cells 30 min after the chemical stimuli. Temperature mapping in a different cell line With the method established in this study, intracellular temperature imaging was also performed in living HeLa cells. The functionality of FPT was confirmed in a HeLa cell extract ( Supplementary Fig. S13 ) and in living HeLa cells ( Supplementary Fig. S14 ). Intracellular temperature imaging in HeLa cells indicated the higher temperature of the nucleus ( Supplementary Fig. S15 ), the centrosome ( Supplementary Fig. S16 ) and mitochondria ( Supplementary Fig. S17 ), as seen in the imaging of COS7 cells. The results demonstrating the temperature gradient in both living HeLa and COS7 cells display the universal characteristics of our findings among mammalian cells. In this study, we have established a method for imaging the temperature distribution inside living cells by performing TCSPC-FLIM of our novel FPT. By exploiting the high spatial resolution of FPT, intracellular temperature imaging revealed the thermal profiles of living cells, that is, the higher temperatures of the nucleus, centrosome and the areas near the mitochondria. Recently, numerous temperature sensors have been developed to meet the urgent demand for measuring temperature in a tiny intracellular space. Among these emerging thermometers, which are based on lanthanide nanoparticles [13] , [16] , [17] , [19] , [20] , dye-coated nanoparticles [14] , quantum dots [15] , semiconducting polymer dots [18] and temperature-responsive polymers [21] , [22] , FPT in this study is the only thermometer that allows the mapping of intracellular temperatures due to its ability to diffuse throughout living cells and its sensitivity to temperature. In terms of sensitivity, the intracellular temperature variations unveiled in this study indicated that fluorescent molecular thermometers for intracellular temperature mapping must have the ability to distinguish a temperature difference of less than 1 °C. Related to this requirement, an appropriate evaluation of temperature resolution should be carefully considered for reliable intracellular thermometry (cf. Fig. 2b and Methods). It should also be noted that a fluorescence response of FPT to temperature change was observed in the range of 20–50 °C ( Fig. 1c, d ), which was much wider than that of our previous thermometer, FNT (27–33 °C). This is a bonus property of FPT. Consequently, the intracellular temperature of a wider range of subjects can be measured using our present thermometry. In addition to our novel FPT, the TCSPC-FLIM technique also contributed to the realization of intracellular temperature mapping with high spatial and temperature resolution. In measuring local intracellular temperature that differed among sub-cellular locations, the fluorescence intensity of a fluorescent molecular thermometer was not an appropriate variable for calculating temperature, because it also strongly correlates with the concentration of the fluorescent molecular thermometer. As temperature-dependent but concentration-independent variables, fluorescence lifetime [38] , [39] , maximum emission wavelength [15] and a ratio of fluorescence intensities at two different wavelengths [10] , [13] , [17] , [18] are all useful. In our methodology, the fluorescence lifetime was chosen because of its high sensitivity and accuracy when the robust TCSPC-FLIM technique was utilized [24] , [40] . Another advantage of the fluorescence lifetime in bio-imaging is multidimensionality [41] . As for FPT, the number of components in the fluorescence lifetime represents the number of states that the fluorophore assumes. TCSPC-FLIM showed that the fluorescence lifetime of FPT consisted of two components in both a cell extract and a living cell ( Fig. 2a and Supplementary Fig. S7 ), indicating that the DBD-AA units in FPT assumed two defined states (that is, hydrogen-bonded and hydrogen bond-free states) [30] in both aqueous media, and that the interaction between these media and FPT was analogous. Thus, the calibration curve ( Fig. 2b ) obtained using the cell extract was effective for intracellular temperature mapping in living cells. In contrast, single-dimensional variables (that is, maximum emission wavelength and fluorescence intensity ratio) would not allow us to compare the interactions between different environments (that is, in vitro and in vivo in our study) and the fluorophore; hence, the accuracy of thermometry would be compromised. The fluorescence lifetime of FPT in living cells is potentially influenced by changes in environmental viscosity. Here, we indicate that the heterogeneous fluorescence lifetime of FPT in the fluorescence lifetime images of living cells (for example, Figs 3 , 4 and 6 ) did not originate from variations in viscosity. The fluorescence image of FPT dispersed in living COS7 cells ( Fig. 1g ) and the recovery of fluorescence signal in the FRAP (fluorescence recovery after photobleaching) experiments using FPT and living COS7 cells ( Supplementary Fig. S18 ) showed that FPT microinjected into cells could freely move in the cytoplasm and the nucleus without any localization in organelles. Therefore, the variation in viscosity, which may have an effect on FPT in living cells, can be estimated in the range from 0.9 to 1.1 cP (in the cytoplasm) to 1.4 cP (in the nucleus) [42] , [43] , [44] . The fluorescence lifetime measurements of FPT in Ficoll solutions with different concentration (that is, viscosity; Supplementary Fig. S6 ) indicated that the fluorescence lifetime of FPT was almost identical in all concentrations. Because of this functional independency of FPT from the variations in environmental viscosity, the accuracy of our intracellular thermometry was assured. The intracellular temperature map we drew in this study demonstrates the existence of a temperature gradient inside a living cell. Furthermore, this inhomogeneous temperature distribution is intrinsically related to fundamental cellular processes, such as the cell cycle and the stimulation of the mitochondria. Our results are in a good accordance with the study by Zohar et al . [11] , in which temperature imaging of cell surfaces was performed by locating a fluorescent molecular thermometer on the cell membrane, in that both results indicate the spontaneous and significant thermogenesis upon the stimulation of steady-state live cells. In comparison, our methodology of imaging intracellular temperature is of distinct superiority with respect to the sensitivity, the spatial resolution, functional independency and ability to function inside living cells. These findings have a significant impact on the comprehension of cell function in different aspects of molecular and cellular structure, and provide insights into the regulatory mechanisms of intracellular signalling. Therefore, in future, intracellular temperature imaging, relating specifically to various cell species (that is, animal and plant cells in both normal and pathological conditions) and cellular activities (that is, cell division, differentiation, or stress responses) will assist in the study of intracellular thermodynamics and thereby aid future discoveries of the profound mechanisms of life. Preparation of FPT and the control copolymer NNPAM [45] (2.4375 mmol), SPA(62.5 μmol, Aldrich), DBD-AA(25 μmol) [26] and α,α′-azobisisobutyronitrile (25 μmol) were dissolved in N , N -dimethylformamide (5 ml), and the solution was bubbled with dry nitrogen for 30 min to remove dissolved oxygen. The solution was heated to 60 °C for 12 h and then cooled to room temperature. The reaction mixture was then poured into diethyl ether (200 ml). The obtained FPT was purified by reprecipitation using methanol (3 ml)–diethyl ether (200 ml) and dialysis (yield: 35%). For the preparation of the control copolymer, N -ethylacrylamide (NEAM, 2.4375 mmol, Monomer-Polymer & Dajac Labs) was used instead of NNPAM (yield: 16%). The contents of the NNPAM, NEAM and SPA units in the copolymers were determined from 1 H-nuclear magnetic resonance spectra (Bruker AVANCE400). The proportions of the DBD-AA units in the copolymers were determined from their absorbance in methanol compared with the model fluorophore N ,2-dimethyl- N -(2-{methyl[7-(dimethylsulfamoyl)-2,1,3-benzoxadiazol-4-yl]amino}ethyl)propanamide (DBD-IA) [30] ( ɛ =10,800 M −1 cm −1 at 444 nm). The molecular weights of the copolymers were determined using gel permeation chromatography. A calibration curve was obtained using a polystyrene standard, and 1-methyl-2-pyrrolidinone containing LiBr (5 mM) was used as the eluent. The hydrodynamic diameter of FPT (0.001 w/v% in water) was estimated by a dynamic light-scattering measurement at 40 °C with a Zetasizer Nano ZS (Malvern). Fluorescence lifetime measurements in cell extracts The fluorescence lifetime of FPT (or the control copolymer) was measured using a FluoroCube 3000U (Horiba Jobin Yvon) ( Fig. 2c , Supplementary Figs S4–S6 ) or a TCSPC system SPC830 (ver. 3.0, Becker & Hickl) with a TCS SP5 confocal laser-scanning microscope (Leica; Fig. 2a,b,d , Supplementary Figs S9 and S13 ). For the measurements with the FluoroCube, the sample was excited with a pulsed diode laser (NanoLED-405L, Horiba, 405 nm) at a repetition rate of 1 MHz, and the emission from 554 to 566 nm was collected. The temperature of the sample was controlled by an ETC-273T controller (JASCO). The obtained fluorescence decay curve was fitted by a double exponential function: Then, the fluorescence lifetime ( τ f ) was calculated using the following equation: For the measurements with the SPC830, 200 μl of the sample (0.02 w/v%) was excited in a 35-mm glass base dish (No. 3911–035, ASAHI Techno GLASS) with a pulsed diode laser (LDH-P-C-405B, PicoQuant, 405 nm) at a repetition rate of 20 MHz, and the emission from 500 to 700 nm was collected through an HCX PL APO Ibd.BL 63×1.4 NA oil objective (Leica Microsystems) in a 64×64 pixel format. The sample temperature was controlled using a GSI-H1R stage with an INUB-F1 controller (Tokai Hit), and monitored with a thermocouple (TSU-0125 thermometer with a TSU-7225 probe, Tokai Hit). The fluorescence lifetime data were collected for 60 s and analysed using the SPCImage software (Becker & Hickl) with the binning procedure (factor: 5 or 6). The fluorescence lifetime for each pixel was calculated using equation (2) and averaged within the whole image. The calibration curve for the temperature imaging of COS7 cells with FPT was obtained by approximating the relationship between the averaged fluorescence lifetime of FPT in a COS7 cell extract (in triplicate) and the temperature to the sixth-degree polynomial (correlation coefficient r =0.998) where T and τ f ( T ) represent the temperature (°C) and the fluorescence lifetime (ns) at T °C, respectively. The temperature resolution (δ T ) of the fluorescent thermometer was evaluated by the following equation: where ∂ T /∂ τ f and δ τ f represent the inverse of the slope in the fluorescence lifetime temperature diagram and the s.d. of the averaged fluorescent lifetime, respectively. Preparation of cell extract The cell pellets (0.5 ml) were collected and resuspended in hypertonic buffer (2.5 ml, containing 0.42 M KCl, 50 mM HEPES (4-(2-hydroxyethyl)-1-piperazineethanesulfonic acid)-KOH, 5 mM MgCl 2 , 0.1 mM EDTA, 20% glycerol, pH 7.8), followed by lysis using a 25-G needle with a syringe and centrifugation (11,000 r.p.m., 15 min, 4 °C). The supernatant was diluted by 40% with water to adjust its KCl concentration to 0.15 M. The adequacy of using the cell extract was assessed by comparing the fluorescence response of FPT in a COS7 cell extract (obtained by fluorescence spectroscopy) with that in living COS7 cells (obtained by epifluorescence microscopy; Supplementary Fig. S2 ). Fluorescence imaging of the cells Microinjection of FPT, the control copolymer and FNT into living cells was performed with Femtojet (Eppendorf), controlled by a micromanipulator (Eppendorf). The fluorescent thermometers were dissolved in an aqueous solution (1 w/v%) containing 80 mM KCl, 10 mM K 2 HPO 4 and 4 mM NaCl. The solution was filtered using an Ultrafree-MC filter (Millipore) and microinjected into the cytoplasm with a glass capillary needle (Femtotips II, Eppendorf). The volume of the injected solution was estimated to be 2 fl. Epifluorescence imaging was performed on an IX70 inverted microscope (Olympus) equipped with an objective lens (×60, UplanApo NA 1.40, Olympus). The temperature of the culture medium was controlled with a stage and a microscope objective lens heater with a controller (Olympus MI-IBC) and monitored using a thermocouple (TSU-0125 thermometer with a TSU-7225 probe, Tokai Hit). A cooled CCD camera (ORCA-ER, Hamamatsu) was used to acquire cell images. The fluorescence images were taken using a sapphire laser (Model 488–30 CDRH, Coherent), a DM505 dichroic mirror (Olympus) and a BA515–550 emission filter (Olympus). The obtained images were analysed using AQUA-Lite ver. 10 (Hamamatsu). Mitochondria, lysosomes, ER and the Golgi apparatus were stained with MitoTracker Deep Red FM (Invitrogen), CellLight BacMam 2.0 for lysosome C10597 (Invitrogen), ER-tracker Red (Invitrogen) and BODIPY TR C5 ceramide complexed to BSA (Invitrogen), respectively, before microinjection of FNT. The organelles and FNT were then imaged by epifluorescence microscopy (at 28–37 °C). Mitochondria and the Golgi apparatus were visualized using a He-Ne laser (GLS5360, 633 nm; Showa Optronics), a 660LP dichroic mirror (Chroma Technology) and a 610/75M emission filter (Chroma Technology). Lysosomes and ER were imaged using a solid-state laser (Compass 315M-100, 532 nm; Coherent), a 565LP dichroic mirror (Chroma Technology) and a 610/75M emission filter. Confocal fluorescence imaging and fluorescence ifetime imaging were performed on a TCS SP5 confocal laser-scanning microscope equipped with a TCSPC module SPC-830 (as described above, except that the emission was collected from 500 to 620 nm in co-visualization of FPT and mitochondria). The fluorescence was captured through an HCX PL APO Ibd.BL 63×1.4 NA oil objective (Leica Microsystems) with 1 ∼ 9 zoom factors in a 1024×1024 pixel format for confocal fluorescence imaging and in a 64×64 pixel format for fluorescence lifetime imaging (for 60 s). The obtained fluorescence decay curve in each pixel was fitted with a double exponential function using SPCImage software (Becker & Hickl) after the binning procedure (factor: 2 or 3). In evaluating the intracellular temperature by FLIM, the cell periphery regions were omitted from the temperature averaging within a cell, because they gave less than the required 1,000 photon count at the peak of the fluorescence decay curve, which is below that required to obtain a reliable fluorescence lifetime [46] (see Supplementary Fig. S19 ). The s.e. in determining temperature from fluorescence lifetime was evaluated from a deviation of averaged fluorescence lifetime in fluorescence lifetime images of different samples (that is, equal to the temperature resolution). The potential maximum error in determining ΔTemperature in living cells (in Figs 4 , 5 , Supplementary Figs S15 and S16 ) was evaluated from a deviation of fluorescence lifetime within a fluorescence lifetime image, which was examined using a cell extract containing FPT. Mitochondria were labelled with MitoTracker Deep Red FM (Invitrogen), and the fluorescence from 645 to 730 nm was collected using confocal microscopy. The chemical stimulus was conducted by quickly adding 100 μl of 2 mM FCCP (Sigma) in phenol red-free culture medium to the studied cells in 1.9 ml of phenol red-free culture medium in a glass base dish. The temperature of the culture medium was maintained at 30.0 °C. Immunofluorescence imaging of γ-tubulin COS7 cells were fixed with 4% paraformaldehyde in PBS (137 mM NaCl, 2.68 mM KCl, 8.10 mM Na 2 HPO 4 , 1.47 mM KH 2 PO 4 , pH 7.7) for 30 min at room temperature, permeabilized with 0.1% Triton X-100 (Wako) in PBS for 30 min at room temperature and blocked with 1% BSA (Sigma-Aldrich) and 0.1% Tween 20 (Pharmacia Biotech) in PBS. Subsequently, the cells were incubated with a mouse monoclonal anti-γ-tubulin antibody (Abcam). The primary antibodies were detected with secondary anti-mouse IgG1 antibodies labelled with Cy5 (Beckman Coulter). After being washed several times with PBS, the cells were imaged with the epifluorescence microscope using GLS5360, a 660LP dichroic mirror and a 700/75 M emission filter (Chroma technology). How to cite this article: Okabe, K. et al . Intracellular temperature mapping with a fluorescent polymeric thermometer and fluorescence lifetime imaging microscopy. Nat. Commun. 3:705 doi: 10.1038/ncomms1714 (2012).